Piezoelectric-nanowire-enabled power source for driving wireless microelectronics Harvesting energy from irregular/random mechanical actions in variable and uncontrollable environments is an effective approach for powering wireless mobile electronics to meet a wide range of applications in our daily life. Piezoelectric nanowires are robust and can be stimulated by tiny physical motions/disturbances over a range of frequencies. Here, we demonstrate the first chemical epitaxial growth of PbZr x Ti 1−x O 3 (PZT) nanowire arrays at 230 °C and their application as high-output energy converters. The nanogenerators fabricated using a single array of PZT nanowires produce a peak output voltage of ~0.7 V, current density of 4 μA cm −2 and an average power density of 2.8 mW cm −3 . The alternating current output of the nanogenerator is rectified, and the harvested energy is stored and later used to light up a commercial laser diode. This work demonstrates the feasibility of using nanogenerators for powering mobile and even personal microelectronics. The search for sustainable micro/nano-powering sources for driving wireless and mobile electronics is an emerging field in today's energy research, which could offer a fundamental solution to the energy needed for driving nanodevices/nanosystems [1] , [2] , [3] . The piezoelectric nanogenerator that converts mechanical energy into electricity was first demonstrated using ZnO nanowire arrays [4] . Following this initial discovery, both direct current [5] , [6] and alternating current [7] ZnO nanogenerators have been developed. In addition, nanogenerators based on GaN nanowires [8] and poly(vinylidene fluoride) nanofibres [9] have shown promising potential for enhancing the nanogenerator performance. Consequently, a worldwide effort has been launched in this regard, forming a new research field in nanotechnology and energy science [10] . The advantage of using nanowires for energy harvesting is their high mechanical robustness and responsiveness to tiny random mechanical disturbances/stimulation. Although the output voltage of nanogenerators has been raised to 1.2 V using an integration of millions of ZnO nanowires for driving a single nanowire-based UV/pH sensor [11] , the output power of the nanogenerators was still too small to power any conventional electronic components, such as laser diodes (LDs). Lead zirconate titanate, PbZr x Ti 1−x O 3 (PZT), is probably the most important piezoelectric material for sensors and actuators, owing to its remarkable piezoelectric performance [12] , [13] . However, the fabrication of PZT thin films [14] and microfibres [15] usually requires high temperatures (~650 °C) to increase the crystallinity [16] , which leads not only to high cost and incompatibility with general fabrication processes but also makes it difficult to integrate with soft materials, even though a transfer technique has been demonstrated recently [17] . Here, we report the first chemical epitaxial growth of vertically aligned single-crystal PbZr 0.52 Ti 0.48 O 3 nanowire arrays on a variety of conductive and non-conductive substrates by hydrothermal decomposition at 230 °C. Alternating current nanogenerators fabricated using the PZT nanowire arrays showed outstanding output. Using a rectifying circuit, the output electrical energy of the nanogenerator was stored with capacitors and later used to light up a commercial LD. This is a key step in developing sustainable energy technology for micro/nanosystems. Synthesis and characterization of the PZT nanowire arrays PZT nanowire arrays were grown by a hydrothermal process ( Fig. 1a ). The reaction equations are given below. During the nucleation and growth of PZT nanowires, the poly(vinyl alcohol) and poly(acrylic acid) perform as capping agents that chemisorb at the side surfaces of the nanowires and thus inhibit their radial growth. Transmission electron microscopy analysis of a single nanowire ( Fig. 1b and Supplementary Fig. S1 ) and X-ray diffraction of nanowire arrays ( Fig. 1c ) show that the as-synthesized nanowires have a tetragonal phase of single crystalline PZT (space group P4mm) and a [001] growth direction [18] . The vertical growth and alignment were enforced by the epitaxial growth on the inorganic substrate, which have a better alignment than the nanofibres fabricated by electrospinning [15] . A piezoelectric domain boundary was found in the axial direction of the nanowire, but the entire nanowire preserves a single crystal structure ( Supplementary Fig. S1c ). 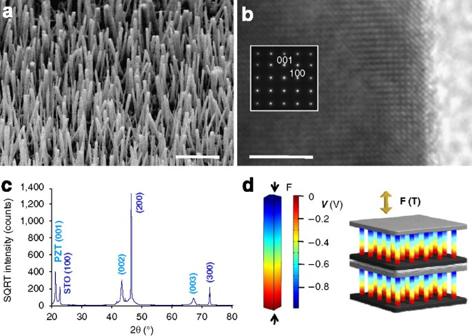Figure 1: PZT nanowire characterization and nanogenerator simulation. (a) Scanning electron microscopy image of the epitaxially grown PZT nanowire arrays on an Nb-doped STO substrate by hydrothermal decomposition. Scale bar, 5 μm. (b) High-resolution TEM image and electron diffraction pattern (inset) acquired from an as-grown PZT nanowire, indicating a well-crystallized tetragonal phase with a lattice constant ofa=3.93 Å andc=4.16 Å. Scale bar, 5 nm. (c) Conventional θ−2θ scan X-ray diffraction spectrum from the as-grown nanowire arrays. (d) Finite element calculation (left) of the piezoelectric potential distribution (~1 V) in a PZT nanowire (d33=1.52×10−10C/N) of 500 nm in width and 5 μm in length, under a uniaxial compression of 2.5 μN. The right-hand side schematic diagram is the structure of a multilayered nanogenerator fabricated using the nanowire arrays. SQRT indicates square root. Figure 1: PZT nanowire characterization and nanogenerator simulation. ( a ) Scanning electron microscopy image of the epitaxially grown PZT nanowire arrays on an Nb-doped STO substrate by hydrothermal decomposition. Scale bar, 5 μm. ( b ) High-resolution TEM image and electron diffraction pattern (inset) acquired from an as-grown PZT nanowire, indicating a well-crystallized tetragonal phase with a lattice constant of a =3.93 Å and c =4.16 Å. Scale bar, 5 nm. ( c ) Conventional θ−2θ scan X-ray diffraction spectrum from the as-grown nanowire arrays. ( d ) Finite element calculation (left) of the piezoelectric potential distribution (~1 V) in a PZT nanowire ( d 33 =1.52×10 −10 C/N) of 500 nm in width and 5 μm in length, under a uniaxial compression of 2.5 μN. The right-hand side schematic diagram is the structure of a multilayered nanogenerator fabricated using the nanowire arrays. SQRT indicates square root. Full size image Fabrication and characterization of the nanogenerator Finite element calculations are used based on a cantilever model that has one end fixed and the other end free. We have three main assumptions. First, the elastic modulus of the nanowire is isotropic and the piezoelectric efficient is anisotropic; second, the nanowire is under pure axial compression and free of shear strain; and third, the piezoelectric domains are all perfectly aligned. The calculation result shows that, for a tetragonal PZT nanowire growing along [001] direction with a 500 nm diameter and 5 μm length, a uniaxial force of 2.5 μN can create a piezoelectric potential (piezopotential) of ~1 V ( Fig. 1d ). To use this high piezopotential, nanogenerators were fabricated using the PZT nanowire arrays grown on conductive Nb-doped SrTiO 3 (STO) substrates [19] , following the schematic shown in Figure 1d . Electrical polarization was required to align the piezoelectric domains in the same direction and in all the nanowires. In the as-grown nanowires, the dipole moments resulting from the position shift of the Ti 4+ /Zr 4+ ions could take six possible orientations along <001>. An electric poling of the nanowires was made by applying an external electric field of 100 KV cm −1 in a dielectric fluid of high dielectric strength, and with the top electrode being negative and bottom electrode positive. As a result, a macroscopic piezoelectric polarization was forced to align upwards, normal to the substrate ( Supplementary Fig. S2 ) [20] . When the PZT nanowires are subject to a uniaxial compressive force, a piezoelectric field is created inside the nanowires, which produces a transient flow of free electrons in the external load to screen the piezopotential. When the force is lifted, the piezopotential diminishes and the accumulated electrons are released. A dynamically applied stress drives the electrons in the external circuit to flow back and forth, resulting in an alternating output. 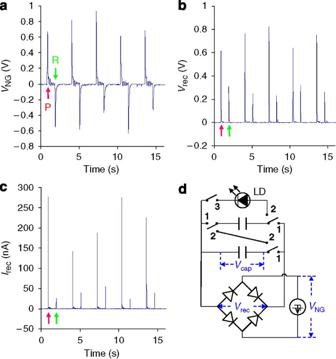Figure 2: Rectification and electrical outputs. (a) Open circuit voltage of a seven-layer integrated nanogenerator before rectification, and (b) open circuit voltage and (c) short circuit current of the nanogenerator after rectification, wherein the outputs when the nanogenerator was compressed and released are indicated with red and green arrowheads, respectively. The projected surface area of the nanogenerator was 6 mm2. (d) Schematic design diagram of the rectifying circuit and charge storage devices, in which the measured voltages are labelled. P, mechanical pressing; R, mechanical releasing. Shown in Figure 2a is the output voltage profile from a seven-layer integrated nanogenerator under a periodic mechanical pressing and releasing. The output voltage is reduced compared with the calculated result owing to the following reasons. First, the height of the nanowires is non-uniform, and only a few percent of the nanowires are actively generating electricity [5] . Second, the nanowires are not perfectly vertically aligned. Hence, when the nanowires are under compression, shear strain is inevitable. Third is the relatively low remnant polarization after the electric field poling ( Supplementary Fig. S2 ). This could be improved by infiltration of insulating polymers into the spacing of the nanowires, and thus increasing the driving voltage. Figure 2: Rectification and electrical outputs. ( a ) Open circuit voltage of a seven-layer integrated nanogenerator before rectification, and ( b ) open circuit voltage and ( c ) short circuit current of the nanogenerator after rectification, wherein the outputs when the nanogenerator was compressed and released are indicated with red and green arrowheads, respectively. The projected surface area of the nanogenerator was 6 mm 2 . ( d ) Schematic design diagram of the rectifying circuit and charge storage devices, in which the measured voltages are labelled. P, mechanical pressing; R, mechanical releasing. Full size image Application of the nanogenerator to power up a microelectric device To fully use the electrical energy harvested by the nanogenerator in one full cycle of mechanical deformation from both pressing and releasing, a current rectification and energy storage system was implemented using a commercial full-wave bridge rectifier composed of four diodes ( Fig. 2d ), each of which had a threshold voltage of 0.3–0.4 V ( Supplementary Fig. S3a ). The voltage and current outputs of the nanogenerator after rectification are shown in Figure 2b and c , respectively, clearly demonstrating full-wave ­rectification. Next, the generated charge pulses were stored consecutively by connecting eight 22 μF capacitors in parallel, as shown in Figure 2d , with the switches set at position '1'. 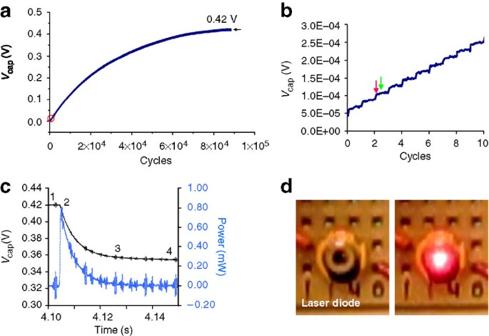Figure 3: Storage of electrical pulses into capacitors to light up a laser diode (LD). (a) Voltage across a storage capacitor when being charged by an alternating current nanogenerator with 0.7 V peak voltage. (b) An enlarged plot of the voltage curve inaat the very beginning of the charging process, as indicated by a red circle. The step increase in capacitor voltage when the nanogenerator is compressed and released is indicated by red and green arrowheads, respectively. (c) Discharging voltage curve across a single capacitor when it was connected in series together with seven other capacitors to a LD (emission wavelength 650 nm, operation power 0.1–6 mW), and the corresponding output power to drive the LD (blue curve).Vcap saturates at 0.42 V (1–2). Then, the capacitors are discharged to light the LD and theVcap drops to 0.35 V (2–3) followed by a slow decay process (3–4). It is suggested that such a discharge behaviour took place when the charges stored in the capacitor were insufficient to light the LD, although the remaining voltage was enough to overcome the LD threshold, though the current was limited. The output power was derived from the discharge curve followingnCVcapdVcap/dt, withn=number of capacitors in serial. The fluctuation in power curve is due to differentiations of the noise in theVcapcurve. (d) Snapshots of the LD before and at the moment of being lit up using the stored charges. See alsoSupplementary Movie 1. The entire charging process was recorded by monitoring the voltage/potential across a capacitor, as presented in Figure 3a . A step increase in the stored energy can be clearly seen with each cycle of the energy conversion process, as indicated by arrowheads in Figure 3b . As the charging process continued, the voltage of the capacitor was saturated to ~0.42 V, which was lower than the peak output voltage of the nanogenerator, possibly due to voltage drop consumed at the rectifying diodes ( Supplementary Fig. S3b ) and/or the leakage of the capacitors, especially when the capacitor voltage was high (see Supplementary Fig. S4 for the charge storage efficiency of the capacitors). Then, by connecting the eight charged capacitors in series by adjusting the switches to position '2' (see Fig. 2d ), the total output voltage reached V tot =0.42×8=3.36 V. This was high enough to drive a LD with a turn-on voltage of ~1.5 V ( Supplementary Fig. S5 ), provided the output power was sufficient at the discharge ( Fig. 3c ). By using this voltage amplification technique, we successfully powered a commercial LD by a fast discharge of the stored charges, as shown in Figure 3d (see Supplementary Movie 1 ). The voltage drop across a capacitor dropped from ~0.42 to ~0.35 V after the discharge process ( Fig. 3c ). This means that ~16.7% of the stored charges was effectively used to drive the LD. The remaining charges were still stored in the capacitor and blocked by the threshold operating voltage of the LD. The next round of charging the capacitors would start at a base voltage of 0.35 V rather than 0 V, thus the following charging cycle should take a lot less time. Figure 3: Storage of electrical pulses into capacitors to light up a laser diode (LD). ( a ) Voltage across a storage capacitor when being charged by an alternating current nanogenerator with 0.7 V peak voltage. ( b ) An enlarged plot of the voltage curve in a at the very beginning of the charging process, as indicated by a red circle. The step increase in capacitor voltage when the nanogenerator is compressed and released is indicated by red and green arrowheads, respectively. ( c ) Discharging voltage curve across a single capacitor when it was connected in series together with seven other capacitors to a LD (emission wavelength 650 nm, operation power 0.1–6 mW), and the corresponding output power to drive the LD (blue curve). V cap saturates at 0.42 V (1–2). Then, the capacitors are discharged to light the LD and the V cap drops to 0.35 V (2–3) followed by a slow decay process (3–4). It is suggested that such a discharge behaviour took place when the charges stored in the capacitor were insufficient to light the LD, although the remaining voltage was enough to overcome the LD threshold, though the current was limited. The output power was derived from the discharge curve following nCV cap d V cap /d t , with n =number of capacitors in serial. The fluctuation in power curve is due to differentiations of the noise in the V cap curve. ( d ) Snapshots of the LD before and at the moment of being lit up using the stored charges. See also Supplementary Movie 1 . Full size image The projected surface area of the nanogenerator used for generating the charges and powering the LD in Figure 3 was ~6 mm 2 . The power generated by such a small nanogenerator cannot drive the continuous operation of a LD. However, an accumulation of charges generated over a period of time is sufficient to drive the LD for a fraction of a second. This can be of practical use for devices that have standby and active modes, such as glucose sensors and blood pressure sensors for health monitoring, or even personal electronics such as bluetooth transmitters (driving power ~5 mW; data transmission rate ~500 kbits s −1 ; power consumption 10 nW per bit) that are only required to be in active mode periodically. The excess energy generated/harvested while the device is in standby is likely sufficient to drive the device when it is in active mode. Frequency dependence of the nanogenerator. The energy storage technique presented here was developed to fully harvest the randomly available mechanical energy for practical applications. The intended use is for harvesting naturally available mechanical agitations rather than a purposely created regular action to drive the nanogenerator. 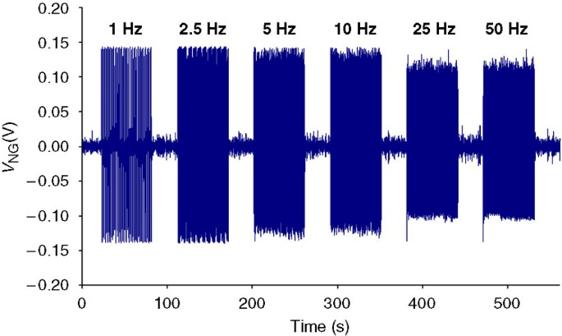Figure 4: Voltage of the nanogenerator as a function of the driving frequency. When the external force frequency is relatively high, the soft packaging epoxy polymer could not respond at the same pace as the external mechanical force, which dampers the magnitude of the external force. Therefore, the amplitude of the output voltage is slightly reduced when the force frequency is increased. Such performance is expected to be improved with the exploration of new packaging materials and technologies. The output voltage of a PZT nanowire-based nanogenerator at a range of stimulating frequencies from 1 to 50 Hz is shown in Figure 4 . This demonstrates that the nanogenerator is able to work at a range of low frequencies, such as human walking, heart beating and vessel contracting, and its capability of powering in vivo biosensors by harvesting biomechanical and/or biofluid hydraulic energies. In addition, the nanogenerators could be configured to work under a relatively high frequency of ~50 KHz [21] . In such a frequency range, the average output power is about half of the peak output power, and thus, an average power density of 2.8 mW cm −3 is conceivable by increasing the agitation frequency shown in Figure 2 . Figure 4: Voltage of the nanogenerator as a function of the driving frequency. When the external force frequency is relatively high, the soft packaging epoxy polymer could not respond at the same pace as the external mechanical force, which dampers the magnitude of the external force. Therefore, the amplitude of the output voltage is slightly reduced when the force frequency is increased. Such performance is expected to be improved with the exploration of new packaging materials and technologies. Full size image In comparison to its thin-film counterparts, PZT nanowires have several figures of merit. First, facial growth of high crystallinity PZT nanowires by wet chemical methods exhibits a great advantage for scaling up at a low cost and the possibility of being transferred onto flexible substrates [17] , whereas single-crystal PZT thin films are fabricated at high temperature using chemical vapor deposition [22] . Second, in comparison with the polycrystalline PZT nanofibres [15] , the single crystalline PZT nanowires have extremely high elasticity and are resistant to fatigue, allowing large degrees of mechanical deformation without fracture [23] . This results in largely enhanced energy conversion efficiencies owing to non-linear mechanical properties. Third, in comparison with polycrystalline PZT bulk and nanostructures [12] , [13] , [15] , the single crystalline PZT nanowires are expected to have higher piezoelectric constants because of the absence of domain boundaries that would pin up the dipole moments. Forth, the force/stress required to induce the mechanical deformation of the nanowires is rather small in comparison with that needed to deform a solid thin-film-based energy harvester, thus permitting nanowire-based nanogenerators to operate in scenarios where only small triggering forces are available, such as in biological system, tiny vibration and even small pressure fluctuation [24] . Finally, the nanogenerators based on nanowires do not require a specific driving frequency to operate, but can be driven by a wide range of irregular/random low-frequency mechanical agitations that are abundant in our daily life. In contrast, the thin-film-based cantilever energy harvesters only work at their high resonant frequencies and harmonics [25] , which may not be ideal for application in our living environment of irregular physical motion and time-dependent variant amplitudes. In conclusion, epitaxial growth of PbZr 0.52 Ti 0.48 O 3 nanowire arrays by a hydrothermal decomposition at 230 °C has been demonstrated for the first time, opening the possibility of low-temperature epitaxial growth of PZT nanowire arrays by wet chemical approaches. Nanogenerators made using a single layer of PZT nanowire arrays gave an output peak voltage of ~0.7 V, peak current density of 4 μA cm −2 and an average power density of 2.8 mW cm −3 , which is 6–12 times higher than that of PZT cantilever [26] , [27] . By using a rectifying circuit, the electrical energy from a seven-layer integrated nanogenerator was rectified and stored into capacitors, which was then used to light up a commercial LD. This is a milestone in achieving the goal of applying nanowire nanogenerators for future self-powered, wireless nanodevices and even personal microelectronics. Growth of PZT nanowire arrays Conductive substrates, 0.7 wt% Nb-doped STO (100) and 0.01 wt% Fe-doped STO (100) (~0.007 Ω cm), were chosen for the epitaxial growth owing to their small lattice mismatch with PZT ( Fig. 1a ). The growth solution (50 ml) was prepared by mixing 0.8168 g (C 4 H 9 O) 4 Ti dissolved in 26 ml ethanol, and 0.8379 g ZrOCl 2 ·8H 2 O dissolved in 30 ml de-ionized water [28] , [29] . Then the Ti 4+ ethanol solution was added drop by drop into the Zr 4+ aqueous solution under vigorous stirring. The mixed solution was introduced into 150 ml of 0.25M NH 3 ·H 2 O, resulting in a white precipitation of Zr 0.52 Ti 0.48 O(OH) 2 . After filtering and rinsing to get rid of the residual Cl − , NH 3 ·H 2 O, C 4 H 9 OH and C 2 H 5 OH, the white precipitate Zr 0.52 Ti 0.48 O(OH) 2 was redispersed in distilled water. Under vigorous stirring, 1.656 g Pb(NO 3 ) 2 , 5.611 g KOH, 0.02 g poly(vinyl alcohol) and 0.36 g poly(acrylic acid) were consecutively added. Next, the hydrothermal solution was placed inside a stainless steel autoclave with a Teflon liner and with the substrate leaning against the sidewall. It was then placed in an oven at 230 °C for 12 h. The final product was baked at 60 °C for 2 h. Fabrication and measurement of the nanogenerator A piece of Si wafer was coated consecutively with layers of 50 nm Ti and 300 nm Pt by electron beam evaporation. The Pt side of the Si wafer was placed on top of the nanowire arrays to form an intimate electrical contact. Each layer was a distinct nanogenerator, with each set of two terminals insulated from the other layers, and the entire structure was packaged with soft epoxy polymer to ensure the robustness of the device and also isolate possible moisture erosion to the nanowires. The area of the nanogenerator layer was ~6 mm 2 . Three-dimensional integration of the nanogenerators was accomplished by stacking multiple layers of the described structure. In our study, the as-fabricated alternating current nanogenerator was measured by the dynamic mechanical stimulation triggered by a linear motor that provided a controllable impact speed, force and frequency. How to cite this article: Xu, S. et al . Piezoelectric-nanowire enabled power source for driving wireless microelectronics. Nat. Commun. 1:93 doi: 10.1038/ncomms1098 (2010).